Microlens arrays in the complex visual system of Cretaceous echinoderms It has long been assumed that photosensitivity in echinoderms is mainly related to diffuse photoreception mediated by photosensitive regions embedded within the dermis. Recent studies, however, have shown that some extant echinoderms may also display modified ossicles with microlenses acting as sophisticated photosensory organs. Thanks to their remarkable properties, these calcitic microlenses serve as an inspiration for scientists across various disciplines among which bio-inspired engineering. However, the evolutionary origins of these microlenses remain obscure. Here we provide microstructural evidence showing that analogous spherical calcitic lenses had been acquired in some brittle stars and starfish of Poland by the Late Cretaceous (Campanian, ~79 Ma). Specimens from Poland described here had a highly developed visual system similar to that of modern forms. We suggest that such an optimization of echinoderm skeletons for both mechanical and optical purposes reflects escalation-related adaptation to increased predation pressure during the so-called Mesozoic Marine Revolution. Among echinoderms, discrete photoreceptive organs with putative image-forming capacity are only known to date in some starfish and one sea cucumber species [1] , [2] , [3] . However, some other echinoderms display a wide range of different behavioural and physiological responses to light [4] , [5] , [6] , [7] . Despite the lack of any direct evidence, the photosensitivity of these animals has long been alleged to ‘diffuse’ dermal photoreceptors capable to detect the overall variation in the illumination level [8] . However, there have been major recent advances in our understanding of photoreceptor cells in echinoderms, thanks to the genome sequencing of the purple sea urchin Strongylocentrotus purpuratus [9] , [10] . Latter studies evidenced a unique system of photoreceptors in sea urchin tube feet: its compact skeleton deploys numerous compound eye units acting as a whole as a screening device. Such a network of eye units provides the sea urchin with a directional vision. Recently, compound eyes devoid of true optics enabling low-resolution vision were documented in starfish species [3] . In addition to diffuse photoreceptors embedded within soft tissues, ocular microstructures, conceivably with the function of a compound eye, have also been reported in some brittle stars. For instance, extant photosensitive Ophiocoma wendtii displays calcitic ossicles with optically clear spherical microstructures and migrating screening pigments both acting, respectively, as sophisticated lenses and filters [11] . Such calcitic microlenses display unusual optical properties directing and focusing the light on the underlying neural receptors [12] . Similar lens-like microstructures (probably with the same function), the so-called ‘glassy tubercles’, were observed in some recent starfish species [13] , [14] . Surprisingly, despite an extensive fossil record of echinoderms, no study has dealt so far with the fine-scale analysis of lens-like microstructures in fossil echinoderms. Here we report analogous ocular microstructures in Late Cretaceous (Campanian) brittle stars and starfish. Our findings unveil the role of these lens-like microstructures in Late Cretaceous echinoderms and suggest that the complex visual system in echinoderms had been already acquired in the Late Cretaceous. Geologic setting Echinoderm specimens with microlenses were collected from an abandoned quarry in Rzeżuśnia (Southern Poland, coordinates 50°20′10″N, 19°58′16″E; Fig. 1a–c ). This area belongs to the Miechów Trough as part of the so-called Szczecin–Łódź–Miechów synclinorium [15] . The exposed Cretaceous sequence comprises nearly 20 m of Upper Campanian (~79 Ma) opoka (=calcarenite), marls and cherts [16] , [17] . 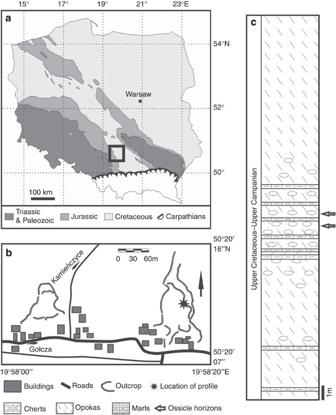Figure 1: Location map. (a) Schematic geological map of Poland and location of investigated area. (b) Outcrop location within investigated area. (c) Schematic lithological section of the Upper Campanian sediments (zones:Inoceramus azerbaydajensis-I. vorhelmensis,Patagiosites stobaei/Galeola basiplanaandGalerites vulgaris/Galeola basiplana17) exposed in the Rzeżuśnia Quarry, arrows=sample location. Figure 1: Location map. ( a ) Schematic geological map of Poland and location of investigated area. ( b ) Outcrop location within investigated area. ( c ) Schematic lithological section of the Upper Campanian sediments (zones: Inoceramus azerbaydajensis-I. vorhelmensis , Patagiosites stobaei/Galeola basiplana and Galerites vulgaris/Galeola basiplana [17] ) exposed in the Rzeżuśnia Quarry, arrows=sample location. Full size image Morphology and microstructure of brittle star plates A lens-like microstructure is observed on the aboral surfaces of 17 brittle star and starfish ossicles. The available brittle star plates consist of radial shields and lateral arm plates (LAPs), tentatively assigned to Stegophiura ? of the family Ophiuridae [18] , [19] ( Fig. 2a–c ). The isolated radial shields are generally robust, triangular and with rounded edges. Their surface comprises an array of closely packed hemispheres ( Fig. 3d,f ). These are the upper halves of almost spherical calcite structures that are relatively uniform in size and shape ( Table 1 ), and are very similar to the lenses in the extant photosensitive species O. wendtii ( Fig. 3a–c , Table 1 ). LAPs are also robust and massive, especially in the most proximal part. Their articulation spurs are weakly developed and hardly visible near the distal edge of the inner surface. Their distal margins display at least nine spine articulations that are relatively high, protruding and bilobate. Of these lobes, the first (probably dorsal) one is massive and bulge-like while the other one (probably ventral) is much thinner and surrounds the muscle opening slightly elongated ventro-distally. These isolated LAPs show a remarkable lens-like ornamentation similar to those of the radial shields ( Fig. 3e ). The lens diameters in Cretaceous and extant brittle stars cannot be statistically segregated from each other (the parametric t -test reports a probability of P >0.05 ( n =20) for equality of the means of lens diameter, giving a non-significant difference). 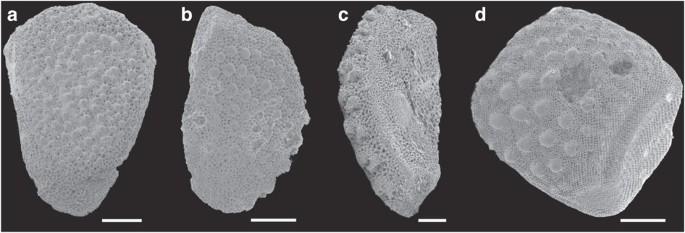Figure 2: Isolated ossicles of brittle stars and of starfish from the Upper Campanian (Upper Cretaceous) of Poland. The images are scanning electron micrographs (SEM). (a) Radial shield ofStegophiura? (dorsal view). (b) Lateral arm plate (LAP) ofStegophiura? (dorsal view). (c) LAP ofStegophiura? (inner-oblique view). (d) Starfish marginal plate (dorsal view). Scale bar, 500 μm. Figure 2: Isolated ossicles of brittle stars and of starfish from the Upper Campanian (Upper Cretaceous) of Poland. The images are scanning electron micrographs (SEM). ( a ) Radial shield of Stegophiura ? (dorsal view). ( b ) Lateral arm plate (LAP) of Stegophiura ? (dorsal view). ( c ) LAP of Stegophiura ? (inner-oblique view). ( d ) Starfish marginal plate (dorsal view). Scale bar, 500 μm. 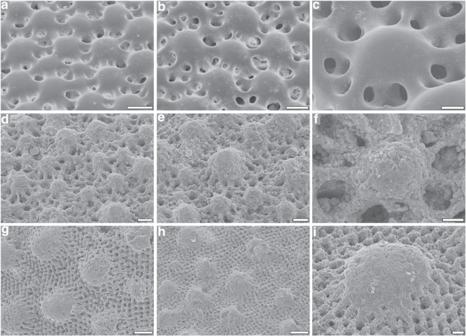Figure 3: Skeletal lens-like microstructure of extant and fossil echinoderms. The images are scanning electron micrographs (SEM). (a) Dorsal arm plate (DAP) ofO. wendtii. (b) Lateral arm plate (LAP) ofO. wendtii(c) Single lens ofO. wendtii. (d) Radial shield of Late Cretaceous brittle starStegophiura? (e) LAP of Late Cretaceous brittle starStegophiura? (f) Single lens of the Late Cretaceous brittle starStegophiura? (g,h) Marginal plate of Late Cretaceous starfish. (i) Single lens of the Late Cretaceous starfish. Scale bar, 50 μm (a,b,d,e), 25 μm (c,f,i) and 100 μm (g,h). Full size image Figure 3: Skeletal lens-like microstructure of extant and fossil echinoderms. The images are scanning electron micrographs (SEM). ( a ) Dorsal arm plate (DAP) of O. wendtii . ( b ) Lateral arm plate (LAP) of O. wendtii ( c ) Single lens of O. wendtii . ( d ) Radial shield of Late Cretaceous brittle star Stegophiura ? ( e ) LAP of Late Cretaceous brittle star Stegophiura ? ( f ) Single lens of the Late Cretaceous brittle star Stegophiura ? ( g , h ) Marginal plate of Late Cretaceous starfish. ( i ) Single lens of the Late Cretaceous starfish. Scale bar, 50 μm ( a , b , d , e ), 25 μm ( c , f , i ) and 100 μm ( g , h ). Full size image Table 1 Comparison of lens diameters in fossil and extant echinoderms. Full size table Morphology and microstructure of starfish plates The starfish ossicles are represented by various marginal plates ( Fig. 2d ). They mostly resemble those observed in Goniasteridae and Benthopectinidae [20] , [21] : they are rather small, robust and blocky. Their outer faces are slightly curved, whereas the lateral faces are parallel to each other, vertical and slightly concave. In these starfish ossicles, the labyrinthic stereom with 10–15 μm thick trabeculae and irregular pores extends into a regular array of lens-like spherical microstructures ( Fig. 3g–i ). The diameter of these probable lenses ( Table 1 ) falls within the range of glassy tubercles in living starfish (30–150 μm) [13] . Although similar oval tubercles (but never interpreted as ocular lenses) have been illustrated in other Mesozoic starfish species [22] , [23] , they are mostly made of dense labyrinthic stereom, not compact, imperforated and non-stereomic calcite as observed in the structures interpreted here as lenses. In cross-section, both starfish and brittle star lenses have a regular cone-like shape identical to those observed in living forms ( Fig. 4b,e,h ). 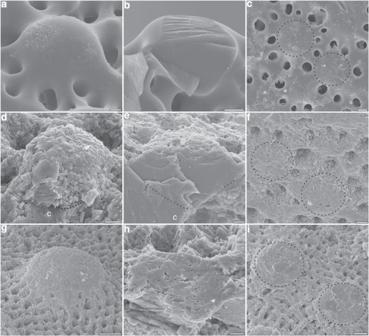Figure 4: Skeletal lens-like microstructures of extant and fossil echinoderms. The images are scanning electron micrographs (SEM). (a) Single lens inO. wendtiiin oblique view. (b) Cross-section of a fractured lateral arm plate (LAP) ofO. wendtiidisplaying an individual microlens. (c) Polished surface of LAP ofO. wendtiishowing the inner structure of individual microlenses (circles). (d) Single lens of the Late Cretaceous brittle starStegophiura? in oblique view. (e) Cross-section of a fractured LAP of a Late Cretaceous brittle starStegophiura? showing an individual microlens. (f) Polished surfaces of LAP of a Late Cretaceous brittle starStegophiura? showing the inner structure of individual microlenses (circles). (g) Single lens of a Late Cretaceous starfish in oblique-lateral view. (h) Cross-section of a fractured marginal plate of a Late Cretaceous starfish showing an individual microlens. (i) Polished surfaces of a marginal plate of a Late Cretaceous starfish showing the inner structure of individual microlenses (circles). Dotted lines indandedelineate the contact between lenses and carbonate cement infills (c). Scale bar, 10 μm (a,b,d,e,h); 50 μm (g); and 20 μm (c,f,i). Figure 4: Skeletal lens-like microstructures of extant and fossil echinoderms. The images are scanning electron micrographs (SEM). ( a ) Single lens in O. wendtii in oblique view. ( b ) Cross-section of a fractured lateral arm plate (LAP) of O. wendtii displaying an individual microlens. ( c ) Polished surface of LAP of O. wendtii showing the inner structure of individual microlenses (circles). ( d ) Single lens of the Late Cretaceous brittle star Stegophiura ? in oblique view. ( e ) Cross-section of a fractured LAP of a Late Cretaceous brittle star Stegophiura ? showing an individual microlens. ( f ) Polished surfaces of LAP of a Late Cretaceous brittle star Stegophiura ? showing the inner structure of individual microlenses (circles). ( g ) Single lens of a Late Cretaceous starfish in oblique-lateral view. ( h ) Cross-section of a fractured marginal plate of a Late Cretaceous starfish showing an individual microlens. ( i ) Polished surfaces of a marginal plate of a Late Cretaceous starfish showing the inner structure of individual microlenses (circles). Dotted lines in d and e delineate the contact between lenses and carbonate cement infills ( c ). Scale bar, 10 μm ( a , b , d , e , h ); 50 μm ( g ); and 20 μm ( c , f , i ). Full size image In contrast with the wide range of calcitic and non-biomineralized microlenses occurring in arthropods [24] , [25] , [26] , [27] , [28] , comparable eye-like structures in echinoderms remained unknown until their discovery in extant photosensitive brittle star species O. wendtii [11] , [29] . As highlighted by Aizenberg and Hendler [12] , thanks to their remarkable optical properties, the brittle star calcitic microlenses offer a high potential for bio-inspired engineering: lightweight, mechanically resistant, aberration free and birefringence free. However, a key question such as the origin of such sophisticated photosensory organs in echinoderms remains unanswered [30] . Although similar oval tubercles are known in Late Cretaceous (mostly Maastrichtian, ~72.1–66 Ma) echinoderms [18] , they were never thoroughly analysed and interpreted as microlenses. Therefore, as a consequence, the present data are indeed the first ones to document this evolutionary innovation and provide a stimulus for a line of future in-depth microstructural investigation of other fossil echinoderms of different age. Despite some diagenetic alteration, the overall morphology of the stereom and microlenses of the ossicles at hand is well preserved and similar to those in living photosensitive relatives. Therefore, in the present state of art and to our knowledge, these fossil specimens represent the earliest so far microanatomical evidence for the occurrence of a highly developed vision in Late Cretaceous echinoderms. Interestingly, it suggests that similar lens-like microstructures occurred in various echinoderm clades in the Late Cretaceous. The question concerning why brittle stars and starfish optimized their skeletons for optical functions is still open. However, it seems probable that the parallel occurrence of these visual systems in Late Cretaceous echinoderms could have been a response to the increased predation pressure during the Mesozoic Marine Revolution [30] , [31] , [32] , [33] . During this period, there was a large-scale diversification of durophagous and grazing predators, such as teleost fishes and decapod crustaceans that is considered to have induced evolutionary changes in benthic marine communities [31] . Our findings highlight the magnitude of anti-predatory innovations already achieved in Late Cretaceous. This predation hypothesis is consistent with recent observations of O. wendtii quickly escaping from predators into dark crevices: a high performance photosensitive organ is highly advantageous in terms of survival in natural habitats [34] . Sample collection During spring and summer 2007 and 2012, several bulk samples of ~25 kg were taken from the middle part of the Upper Campanian section in Rzeżuśnia quarry ( Fig. 1c ). They were processed through up to 10 soaking-and-thawing cycles (lowest temperature ~−19 °C and boiled in a Glauber salt solution). All the samples were then washed and successively sieved (mesh sizes: 1.0, 0.5 and 0.315 mm). The residue material was finally dried at up to ~220 °C. Echinoderm ossicles were picked under a stereoscopic microscope. The studied material is housed at the Department of Earth Sciences, University of Silesia, Poland, under registration numbers GIUS 9-3623/As/1-350. Microstructural analyses of echinoderm skeletons Figured ossicles were photographed with a Phillips XL-20 scanning electron microscope (SEM) at the Institute of Paleobiology of the Polish Academy of Sciences in Warsaw. Lens dimensions were measured directly from SEM photographs. For comparison purpose, the ossicles of a recent photosensitive species O. wendtii from southeastern Florida displaying lens-like microstructure were also SEM investigated. In this case, the soft tissues were removed by soaking in a 5% sodium hypochlorite solution for 24 h at room temperature. The data were statistically analysed using PAST 2.02 software [35] . The lens distribution is not significantly non-normal for any of the ossicles (the Shapiro–Wilk test, P >0.05); thus, we preferably used a parametric t -test for statistical comparison between fossil and extant materials. Nevertheless, the non-parametric Mann–Whitney test also reports a probability of P >0.05 ( n =20) for equality of the medians of lens diameter, giving a non-significant difference. The three-dimensional microstructure of selected ossicles was revealed either in fractures or in thin sections. How to cite this article: Gorzelak, P. et al. Microlens arrays in the complex visual system of Cretaceous echinoderms. Nat. Commun. 5:3576 doi: 10.1038/ncomms4576 (2014).